Diastereodivergent organocatalytic asymmetric vinylogous Michael reactions One of the major challenges of modern asymmetric catalysis is the ability to selectively control the formation of all diastereoisomers of reaction products possessing multiple stereocenters. Pioneers of such diastereodivergent catalytic asymmetric processes have focused on reactions where the newly formed stereogenic centres are proximal to the active carbonyl group. To date, however, diastereodivergent reactions at remote positions remain an unmet challenge. Herein, we describe a catalyst-controlled diastereodivergence in the formation of remote stereocenters in the direct vinylogous Michael reactions of β, γ-unsaturated butenolides to α, β-unsaturated ketones. The reactions are enabled by two complementary, non-enantiomeric multifunctional catalysts, which mutually activate and organise both reactants, affording either the syn- or anti-adduct with high diastereo- and enantioselectivity. These two catalytic systems are also applicable in the Mukaiyama–Michael reactions and tandem Michael–Michael reactions. With the continual advancement of catalytic asymmetric synthesis over the last few decades, increasing numbers of highly diastereo- and enantio-selective reactions affording stereochemically defined products possessing multiple stereocenters have been reported. Commonly, through inherent substrate control, one of the possible diastereomeric products predominates the reaction mixture [1] , and naturally, the absolute stereochemical outcome can be controlled by choice over which enantiomeric form of catalyst is employed. However, over-riding natural substrate diastereoselectivity to bias the formation of the other diastereoisomers still remains a significant challenge [2] . Catalyst-controlled diastereodivergence would be highly desirable to solve this shortcoming and such asymmetric processes could significantly advance the field [3] . Researchers including MacMillan [4] , Deng [5] , [6] , Melchiorre [7] , Maulide [8] , [9] , Carreira [10] , [11] have pioneered diastereodivergent asymmetric catalysis and realized the asymmetric functionalization of α- or β-positions (relative to the active carbonyl group). Controlling the selective formation of remote stereocenters remains a difficult synthetic goal, which has attracted significant attention and resulted in ingenious solutions [12] . However, to date, the application of diastereodivergent catalytic asymmetric strategies to control the selective formation of remote stereocenters in carbon–carbon bond-forming reactions (such as vinylogous Michael reaction) remains elusive. Initially, we wanted to focus our attention on the enantioselective synthesis of γ, γ-disubstituted butenolides from prochiral precursors such as deconjugated butenolides. These compounds contain quaternary stereogenic centres and are important motifs in biologically active natural compounds and medicinally important agents [13] , [14] , [15] , [16] , [17] , [18] . The organocatalytic asymmetric synthesis of γ, γ-disubstituted butenolide derivatives has attracted much attention in the past few years [19] , [20] , [21] , [22] , [23] , [24] , [25] , [26] . However, the key limitation encountered with the previous asymmetric vinylogous reactions using β, γ-butenolides was that only one diastereoisomer was accessed, therefore making it relevant to this study. Herein, we present our development of the first example of a highly diastereodivergent, asymmetric and direct vinylogous Michael reactions of β, γ-unsaturated butenolides to α, β-unsaturated ketones, generating both anti- and syn-adducts by employing complementary, non-enantiomeric primary amine catalytic systems. The catalytic mechanism In an ongoing research programme, we have focused on the development of new primary amine catalysts and their application in asymmetric conjugate addition reactions of various pro-nucleophiles to α, β-unsaturated ketones [27] , [28] , [29] , [30] . We envisaged that variations in the backbones, substituents, connectivity and the presence of additional functionality in different primary amine catalysts could give rise to sufficient differences in the local spatial environment to impact on both diastereo- and enantiocontrol. Particularly, we believed adjusting the nature and size of those groups (such as tertiary amine or secondary amine, hydrogen bond donor) flanking the key primary amine functional group could permit two types of noncovalent interactions: weak and loose, or strong and tight hydrogen-bonding interaction between the catalyst and reactant. A weak and loose H-bonding interaction can direct one of the reactants, while the steric hindrance between two reactants dominates the stereoselectivity. A strong and tight H-bonding interaction can preferentially control the position and orientation of the reactive nucleophilic entity, lower the energy barrier coming from steric hindrance of two reactants and produce the diasteromer which is normally inaccessible. From this, the stereoselective discrimination of the reaction partners and anticipant modulation of the diastereo- and enantioselectivity of the Michael reaction could be realized ( Fig. 1 ). Our aim was to develop two complementary, non-enantiomeric, multifunctional primary amine catalytic systems possessing different skeletal constructs to obtain anti- or syn-products in high enantio- and diastereoselectivities across a range of reaction types. 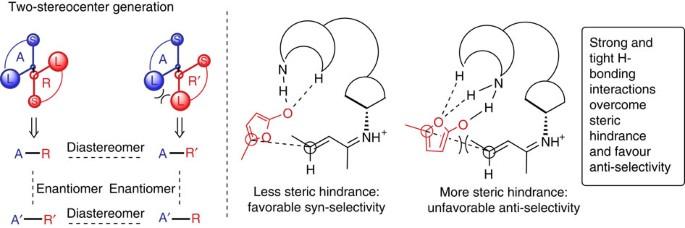Figure 1: The catalytic mechanism. The designed concepts for the diastereodivergent catalytic asymmetric vinylogous Michael reactions with multifunctional catalysts. Figure 1: The catalytic mechanism. The designed concepts for the diastereodivergent catalytic asymmetric vinylogous Michael reactions with multifunctional catalysts. Full size image Optimization of anti-selective Michael reaction conditions To probe the feasibility of catalyst-controlled diastereodivergence in the direct Michael addition of β, γ-unsaturated butenolides and α, β-unsaturated ketones, we investigated as a model reaction the addition of γ-phenyl-butenolide 2a and 3-hepten-2-one 1a employing a range of primary amine catalysts (at 10 mol% loading) in the presence of 20 mol% of benzoic acid. First, we investigated a series of chiral primary amine catalysts ( Table 1 ). The observed anti/syn-selectivities employing three common primary amine catalysts 5 , 6 and 7 (entries 1–3) ranged from 25/75 to 58/42, hence providing proof of concept. Subsequently, two diamines derived from L -tert-leucine (catalysts 8 and 9 ) were screened. The best result of diastereomeric ratio (d.r.) (84/16, entry 4) suggested that a primary amine possessing a vicinal secondary amine permitting strong and tight H-bonding interaction with β, γ-unsaturated butenolides (for example, catalyst 8 ) might be a suitable catalyst construct for anti-selectivity. Then, catalysts 10a–d with the same scaffold of a primary amine, a vicinal secondary amine and sulphonamide as a terminal hydrogen bond donor were tested (entries 6–9). We hoped that the three functional groups could generate the spatially defined chiral pocket necessary to govern both diastereo- and enantiocontrol. Fortunately and very pleasingly, these experiments provided the anti-adduct in excellent enantioselectivities (97–99% enantiomeric excess (e.e.)) with d.r. up to 91/9. The diastereoselectivity of the reaction was observed to be greatly dependent on the steric hindrance around the primary amine group. Certain parameters were adjusted and optimised ( Supplementary Table 1 ), including the change of the solvent (from CH 2 Cl 2 to CHCl 3 ) and acidic additives (from benzoic acid to 2-nitrobenzoic acid), to achieve 71% conversion after 24 h reaction time, 97/3 d.r. and 99% e.e. (entry 10). Table 1 Screening studies of anti-selective Michael reactions of 1a and 2a. 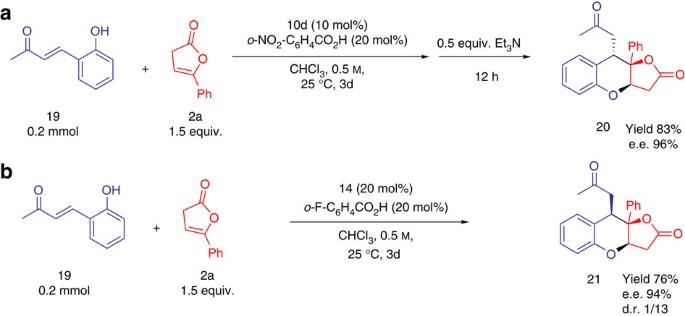Figure 2: Catalyst-controlled enantioselective diastereodivergent tandem Michael–Michael reactions. (a) Catalyzed by catalyst10d, (b) catalyzed by catalyst14. Full size table Optimization of syn-selective Michael reaction conditions After optimization of the conditions for anti-selectivity, the approach for obtaining the other syn-diastereoisomer was further investigated ( Table 2 ). In our initial study, we noted a significant enantioselectivity and reversed diastereoselectivity when catalysts 5 and 6 were employed ( Table 1 , entries 1 and 2). The role of one of the primary amine groups of catalyst 5 and 6 is to activate the enone through generation of an iminium intermediate. It is likely that the other primary amine controls the direction of the nucleophile’s attack by hydrogen-bonding interactions. Accordingly, catalysts derived from diamines 5 and 6 with enhanced hydrogen bond donation ability were conceived to enhance performance. Table 2 Screening studies of syn-selective Michael reactions of 1a and 2a. Full size table Bifunctional primary amine-thiourea catalysts 11 , 12 , 13 and 14 were applied to the model reaction without acidic additives. Good diastereoselectivities (28/72 to 6/94 d.r.) and enantioselectivities (up to 89% e.e.) were obtained (entries 1–4, Table 2 ). Reactivity, as indicated by conversion after 24 h, was disappointing in entries 5–6 when 10 mol% of catalyst 14 and 10 mol% or 20 mol% of benzoic acid was employed as the catalytic system; however, enantioselectivity was marginally improved. After altering a number of the reaction parameters ( Supplementary Table 2 ), including the acid co-catalyst (from benzoic acid to 2-fluorobenzoic acid, entry 7), extending the reaction time (from 24 h to 72 h) and increasing the catalyst and acid additive loading (20 mol%, entry 8), an ideal result of 82% conversion, 6/94 d.r. and 97% e.e. was finally achieved. 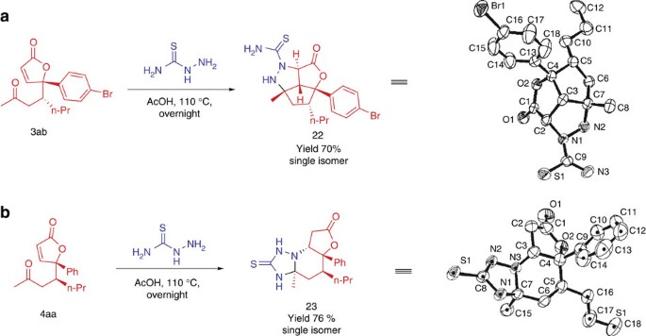Figure 3: Derivatization of the Michael addition products. (a) 1,3-Dipolar cycloaddition of adduct3ab. (b) Tandem reaction of4aa. Substrate scope of anti-selective Michael reaction After the optimal reaction conditions were separately established, the scope of the reaction was investigated as shown in Table 3 , using 10d as the optimal catalyst for anti-selectivity. Table 3 Scope of the Michael reaction for the anti-diastereoisomers 3. Full size table With ( E )-hept-3-en-2-one as the Michael acceptor, a broad range of γ-substituted butenolides, bearing both alkyl substituents and electron-rich/deficient aryl substituents, were investigated. The corresponding anti-products were obtained in good yields with excellent enantio- and diastereoselectivities ( Table 3 , entries 1–8). A butenolide with two alkyl substituents ( Table 3 , entry 9) gave slightly better enantioselectivities than a singly substituted one ( Table 3 , entry 6). Pleasingly, with 5-phenylfuran-2(3 H )-one as the pro-nucleophile, a wide range of enone Michael acceptors bearing various alkyl substituents were reactive and found to give good yields, excellent enantio- and diastereoselectivities ( Table 3 , entries 10–17). Furthermore, other (random) combinations of different γ-substituted butenolides and enones also performed well ( Table 3 , entries 18–23). Reactions of a variety of γ-substituted butenolides and benzalacetone derivatives also proceeded smoothly giving uniformly excellent enantioselectivities, regardless of the position and electron-donating or electron-withdrawing nature of the substituent on the aromatic ring ( Table 3 , entries 24–32). However, with respect to the diastereoselectivity, the result varies with the type of substituent at the γ-position of the butenolides; those with alkyl groups ( Table 3 , entries 27–29, 31–32) performed relatively better than those with an aryl group ( Table 3 , entries 24–26, 30). As for cyclic Michael acceptors, excellent enantioselectivities were observed in moderate-to-good yields; however, 2-cyclopentenone gave a relatively poor diastereoselectivity compared with 2-cyclohexenone or 2-cycloheptenone ( Table 3 , entries 33–37). Taken altogether, our results demonstrate that catalyst 10d is broadly applicable in the anti-selective direct vinylogous Michael addition reaction. Substrate scope of syn-selective Michael reaction As indicated in Table 2 , the syn-diastereoisomer can be obtained under the control of catalyst 14 . To give a clear comparison with the anti-selective reaction described above, the performance of catalyst 14 using exactly the same substrates as in Table 3 were investigated, and the results are summarized in Table 4 . Table 4 Scope of the Michael reaction for the syn-diastereoisomers 4. Full size table With ( E )-hept-3-en-2-one as the Michael acceptor, γ-substituted butenolides bearing electron-rich and -deficient aryl substituents, were investigated in this reaction. The corresponding syn-configured products were observed in moderate yields with good enantioselectivities and diastereoselectivities (from 1/11 to <1/19 d.r.) ( Table 4 , entries 1–4). Unexpectedly, results shown in entries 4–9 in Table 4 turned out to be disappointing under the optimized reaction conditions. After a simple screening of acidic additives ( Supplementary Table 3 ), it was found that the absence of acidic additives would determine moderate yields with excellent enantio- and diastereoselectivities. Doubly alkyl-substituted butenolides gave similar results as those obtained with singly alkyl-substituted butenolides ( Table 3 , entry 9). With 5-phenylfuran-2(3 H )-one as the pro-nucleophile, reactions with enones bearing various short, long or branched chain alkyl groups afforded the corresponding syn-adducts in satisfactory yields with good enantioselectivities and moderate to high diastereoselectivities (from 1/10 to <1/19 d.r.) ( Table 4 , entries 10–17). Different γ-substituted butenolides and enones paired together randomly as shown in Table 4 also gave good enantioselectivities and diastereoselectivities (from 1/15 to <1/19 d.r.) ( Table 4 , entries 18–22). Also, when R 1 substituent was an ethyl group, the corresponding product was obtained in a moderate diastereoselectivity (1/9 d.r.) and yield but with a good enantioselectivity ( Table 4 , entry 23). We found that reaction of γ-phenyl-butenolide and the benzalacetone proceeded poorly in terms of enantioselectivity (55% e.e.) and diastereoselectivity (1/2.7 d.r.). However, by employing 3,5-dinitrobenzoic acid instead of 2-fluorobenzoic as the acidic additive in a more diluted reaction mixture ( Supplementary Table 4 ), satisfactory yields with good enantioselectivities (84–90% e.e.) and better diastereoselectivities (from 1/5 to 1/10 d.r.) could be achieved ( Table 4 , entries 24–26, 30). The reaction of γ-alkyl-butenolides and benzalacetone derivatives proceeded well, efficiently providing the syn-configured products in excellent enantioselectivities and moderate-to-good diastereoselectivities (from 1/6 to 1/13 d.r.) ( Table 4 , entries 27–29, 31–32). The reaction of 2-cyclopentenone (a challenging substrate) and α-angelica lactone resulted in a good enantioselectivity and moderate diastereoselectivity, but a low yield that reflected poor conversion (20% yield after 144 h, Table 4 , entry 33). However, disappointingly, the reaction of 2-cyclopentenone and γ-phenyl-butenolide showed only trace conversion ( Table 4 , entry 34). However, with 2-cyclohexenone as substrate, reactions with both α-angelica lactone and γ-phenyl-butenolide afforded the corresponding syn-configured adducts in moderate yields with excellent enantio- and diastereoselectivities ( Table 4 , entries 35, 36). For the reaction of γ-phenyl-butenolide and the 2-cyclopentenone, the corresponding adducts were obtained in moderate yields with excellent enantioselectivity and moderate diastereoselectivity (1/9 d.r.) ( Table 4 , entry 37). As shown in Table 4 , our results demonstrate a broadly useful method for the synthesis of syn-configured adducts from a wide range of substrates using catalyst 14 . Substrate scope of anti-selective Mukaiyama–Michael reaction After fully establishing the scope of the Michael reaction for both anti- and syn-configured diastereoisomers, we wanted to further examine the possibility of applying the catalyst dual-control strategy in the Mukaiyama–Michael reaction, using γ-substituted- N -Boc-2-(tert-butyldimethylsilyl)oxy-pyrroles 16 as nucleophiles. After adjusting certain parameters ( Supplementary Table 5 ), the optimal reaction conditions for the anti-selective Mukaiyama–Michael reaction were established using catalyst 10c . As shown in Table 5 , with γ-methyl- N -Boc-2-(tert-butyldimethylsilyl)oxy-pyrrole as one substrate, the reaction with various enones was successful and anti-configured products were obtained in moderate yields with good enantioselectivities and moderate diastereoselectivities (from 5/1 to 7/1 d.r.) ( Table 5 , entries 1–3). Using γ-phenyl- N -Boc-2-(tert-butyldimethylsilyl)oxy-pyrrole and benzalacetone as the substrates, an excellent enantioselectivity (96% e.e.) was observed albeit with a poor diastereoselectivity (1.2/1 d.r.) ( Table 5 , entry 4). In this Mukaiyama–Michael reaction, alcohol or H 2 O can accelerate the deprotection of TBS. However, fast deprotection will result in γ-substituted 3-pyrrolidin-2-one without Michael reaction. Table 5 Scope of the anti-selective Mukaiyama–Michael reaction. Full size table Substrate scope of syn-selective Mukaiyama–Michael reaction After certain parameters had been adjusted and the optimal reaction conditions for the complementary syn-selective Mukaiyama–Michael reaction established using catalyst 14 , the same substrate scope of γ-substituted- N -Boc-2-(tert-butyldimethylsilyl)oxy-pyrroles 16 and α, β-unsaturated ketones was probed. As summarized in Table 6 , the corresponding adducts were obtained in moderate-to-good yields with good enantio- and diastereoselectivities (from 1/11 to 1/16 d.r.) ( Table 6 , entries 1–3). Using γ-phenyl- N -Boc-2-(tert-butyldimethylsilyl)oxy-pyrrole and benzalacetone as the substrates, a poor diastereoselectivity (1/1.2 d.r.) was again observed; however, the major anti-configured product was formed with good enantioselectivity ( Table 6 , entry 4). These results demonstrated that our non-enantiomeric catalyst-controlled strategy for diastereodivergence could be applied to the Mukaiyama–Michael reaction of γ-substituted- N -Boc-2-(tert-butyldimethylsilyl)oxy-pyrrole 16 to α, β-unsaturated ketones. Table 6 Scope of the syn -selective Mukaiyama–Michael reaction. Full size table Diastereodivergent tandem Michael–Michael reactions The feasibility of a catalyst-controlled diastereodivergent process in the tandem Michael–Michael reaction also attracted our attention. As demonstrated in Fig. 2 , 5-phenylfuran-2(3 H )-one was reacted with enone 19 (possessing a suitably placed hydroxyl group) under the control of catalyst 10d and subsequently treated with Et 3 N for another 12 h. Diastereoisomer 20 was obtained in a good yield (83%) with excellent enantioselectivity and no other diastereoisomer was detected in the reaction mixture. However, under the control of catalyst 14 the corresponding diastereoisomer, product 21 , was obtained directly and efficiently (76% yield) and with excellent enantioselectivities (94% e.e.) using optimal reaction conditions established above. The relative stereochemical configurations of both products 20 and 21 were established using single-crystal X-ray analysis ( Supplementary Tables 6 and 7 ). Figure 2: Catalyst-controlled enantioselective diastereodivergent tandem Michael–Michael reactions. ( a ) Catalyzed by catalyst 10d , ( b ) catalyzed by catalyst 14 . Full size image Derivatization of the adducts Having successfully extended diastereodivergent processes to a variety of reaction types and a wide range of substrates, we then devoted our efforts to exploring some additional transformations of the enantioenriched and diastereomerically pure Michael addition products, as demonstrated in Fig. 3 . Interestingly, the anti-adduct 3ab was transformed, presumably via a 1,3-dipolar cycloaddition, into an unprecedented [5, 5, 5] tricyclic cage-like compound 22 as a single diastereoisomer when treated with thiosemicarbazide and heated in AcOH at 110 °C overnight. A single crystal of product 22 was subjected to X-ray analysis and established the configuration of 3ab to be R, R ( Supplementary Table 8 ). Interestingly, the syn-adduct 4aa performed differently under the same conditions and was transformed into a complex-fused ring compound 23 via a combination of an aza-Michael addition reaction and an aminoacetalization. Single-crystal X-ray analysis of product 23 established the configuration of 4aa to be R, S ( Supplementary Table 9 ). Figure 3: Derivatization of the Michael addition products. ( a ) 1,3-Dipolar cycloaddition of adduct 3ab . ( b ) Tandem reaction of 4aa. Full size image In short, we have established new methodologies to control the selective formation of remote stereocenters at γ-positions via diastereodivergent catalytic asymmetric processes. We have developed two catalytic systems and investigated their applicability in the asymmetric vinylogous Michael addition of γ-substituted butenolides to α, β-unsaturated ketones. The reactions proceed smoothly with a wide range of substrates and afforded selectively either syn- or anti-configured products, possessing vicinal quaternary and tertiary stereogenic centres, with high enantiocontrol. Furthermore, this approach was applicable to the Mukaiyama–Michael addition of γ-substituted- N -Boc-2-(tert-butyldimethylsilyl)oxy-pyrrole 16 to α, β-unsaturated ketones and also tandem reactions of γ-substituted butenolides with α, β-unsaturated ketone 21 . Both catalytic systems could access major diastereomers with high enantiocontrol but minor diastereomers with low or moderate enantiocontrol. In addition, the different configurations of Michael adducts were diversified further to structure-divergent complex heterocyclic compounds. Studies on further applications of the reported strategy are currently underway and will be reported in due course. General methods For high-performance liquid chromatography charts, 1 H and 13 C nuclear magnetic resonance spectra of compounds in this manuscript, see Supplementary Figs 1–253 . Single-crystal X-ray analysis of catalyst 10c and 14 , see Supplementary Tables 10 and 11 . For details of the synthetic procedures, see Supplementary Methods . Accession codes : The X-ray crystallographic coordinates for structures reported in this Article have been deposited at the Cambridge Crystallographic Data Centre (CCDC), under deposition numbers CCDC-981120 (cat. 10c ), CCDC-981119 (cat. 14 ), CCDC-996776 ( 20 ), CCDC-996772 ( 21 ), CCDC-981117 ( 22 ) and CCDC-981118 ( 23 ). These data can be obtained free of charge from The Cambridge Crystallographic Data Centre via www.ccdc.cam.ac.uk/data_request/cif . How to cite this article: Li, X. et al. Diastereodivergent organocatalytic asymmetric vinylogous Michael reactions. Nat. Commun. 5:4479 doi: 10.1038/ncomms5479 (2014).